Chemo-mechanics of salt damage in stone Many porous materials are damaged by pressure exerted by salt crystals growing in their pores. This is a serious issue in conservation science, geomorphology, geotechnical engineering and concrete materials science. In all cases, a central question is whether crystallization pressure will cause damage. Here we present an experiment in which the crystallization pressure and the pore saturation are varied in a controlled way. We demonstrate that a strain energy failure criterion can be used to predict when damage will occur. The experiment considered is the most widely used means to study the susceptibility to salt crystallization, so quantification of this test has far-reaching implications. The crystallization pressure exerted by salts growing in porous hosts plays a major role in the weathering of materials, in both the natural and built environment. While this was recognized long ago in geomorphology [1] , [2] and conservation science [3] , [4] , [5] , [6] , [7] , it has only recently emerged in concrete science as the most convincing explanation for sulfate attack [8] , [9] , [10] and in geotechnical engineering for the floor heave of anhydrite-containing rock formations [11] . In the latter case, the most dramatic situation was a geothermal drilling through anhydrite-bearing rock formations that opened access for water to convert anhydrite to gypsum. In the neighbouring town, this resulted in a ground uplift of ~26 cm and differential movements causing serious cracking in many buildings [12] . The same process also poses severe issues in tunnelling and mining, causing some tunnels to be periodically closed for rehabilitation because of excessive floor heave [13] . The subject of crystallization pressure has been driven by geomorphology [14] , [15] , [16] , where it is considered to play an important role in the shaping of landscapes, both on Earth [17] and Mars [18] , [19] , [20] . However, it is in conservation science that the consequences of crystallization pressure are most feared because of their impact on monuments, such as the Pharaonic constructions in Luxor [21] , the carved city of Petra [22] , [23] and the medieval city of Rhodes [24] . Crystallization pressure is even more devastating for wall paintings because of the rapid irreversible damage it can cause to works such as Michelangelo’s frescoes in the Sistine Chapel [25] , the tomb of Nefertari [26] , [27] or prehistoric rock art such as the Albarracin Cultural Park [28] , to name only a few. 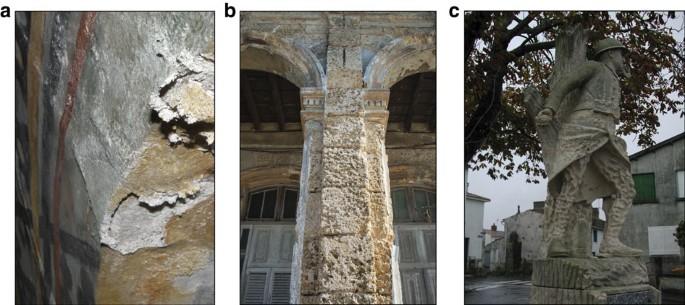Figure 1: Examples of the devastating action exerted by salts. (a) Painted frame of a window in the Valère Basilica in Sion, VS (Switzerland). (b) A column in a building on the Malecón in Havana (Cuba). (c) A statue in La Rochelle (France). Photo a is courtesy of F. Girardet. Photo b is property of the authors. Photo c is by R. van Hees. Figure 1 shows three different examples of the devastating action exerted by salts. Figure 1: Examples of the devastating action exerted by salts. ( a ) Painted frame of a window in the Valère Basilica in Sion, VS (Switzerland). ( b ) A column in a building on the Malecón in Havana (Cuba). ( c ) A statue in La Rochelle (France). Photo a is courtesy of F. Girardet. Photo b is property of the authors. Photo c is by R. van Hees. Full size image Soluble salts accumulate in building materials over years, either because of capillarity, aerosol deposition or reactions of the stone with atmospheric pollutants. It is under specific microclimate conditions that significant crystallization pressures may develop. Research on crystallization pressure has therefore been addressed from quite diverse disciplines that have been mutually enriched, particularly over the past years with their common striving to understand the microscopic origin of weathering processes [29] . This has led to the consensus that salts growing under confined and supersaturated conditions exert crystallization pressure [4] , [16] , [30] , [31] against their porous hosts, subjecting them to tensile stresses. These are particularly damaging for materials with low tensile strength, such as stone (rock), bricks, rammed earth or concrete [31] . However, while much progress has been made in understanding microscale phenomena, a major challenge still remains: predicting under which conditions damage may occur. To address this issue, we examine the experiment most broadly used to study the impact of salt crystallization on materials [7] , [32] , [33] , [34] . Initially proposed in 1828 (ref. 35) [35] , it has undergone minor modifications but continues to rely on cycles of impregnation and drying with a solution containing sodium sulfate, the most devastating salt known [36] . Sodium sulfate and its damaging nature Samples are damaged during impregnation ( Fig. 2 ) because of a phase change from the anhydrate present in the dry state (thenardite, Na 2 SO 4 ) to the decahydrate present in the wet state (mirabilite, Na 2 SO 4 ˙10H 2 O). Thenardite dissolves during impregnation, which creates a high supersaturation with respect to mirabilite that makes it possible for mirabilite to exert a high crystallization pressure during its growth [37] , [38] , [39] , [40] , [41] . No damage is observed during the drying phase [7] . 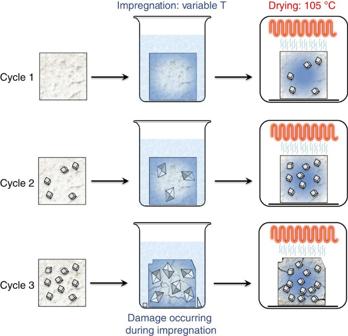Figure 2: Scheme of the sodium sulphate experiment. In the first cycle, the stone fills with sodium sulfate solution. During the drying, sodium sulfate crystallizes as thenardite (cubes). In the subsequent cycle, thenardite converts to mirabilite (octahedrons) through a dissolution–precipitation process made possible by the ingress of sodium sulfate solution. The solution concentration and temperature, as well as the stone strength, determine at which cycle this process will eventually lead the corresponding crystallization pressure to cause damage (mass loss). In this specific example, this is shown already in the 3rd cycle. Figure 2: Scheme of the sodium sulphate experiment. In the first cycle, the stone fills with sodium sulfate solution. During the drying, sodium sulfate crystallizes as thenardite (cubes). In the subsequent cycle, thenardite converts to mirabilite (octahedrons) through a dissolution–precipitation process made possible by the ingress of sodium sulfate solution. The solution concentration and temperature, as well as the stone strength, determine at which cycle this process will eventually lead the corresponding crystallization pressure to cause damage (mass loss). In this specific example, this is shown already in the 3rd cycle. Full size image Sodium sulfate can crystallize in at least eight different crystalline phases. At 20 °C, two are stable and three are metastable. The stable phases are mirabilite (or Glauber’s salt) and thenardite (phase V). The metastable phases are a heptahydrate, Na 2 SO 4 ˙7H 2 O, and two other anhydrous ones (phases III and IV), Na 2 SO 4 . Anhydrous phases I and II exist only at higher temperatures (>270 and >225 °C, respectively), whereas the octahydrate, Na 2 SO 4 ˙8H 2 O, is formed under high-pressure conditions [42] , [43] , [44] , [45] . Until relatively recently, most literature on the subject focused on the two stable phases and generally overlooked the heptahydrate, often stated to form only under laboratory conditions. Experimental investigations by NMR have, however, shown that this is the phase that forms most readily when samples are cooled, and that it persists unless the temperature is brought down close to 0 °C (refs 45 , 46 ). Some studies had suggested that the heptahydrate has very low solid–liquid interfacial energies and is thus incapable of generating high crystallization pressures [47] , [48] . While these statements may be somewhat revised, they remain in general agreement with more recent work by the same group that measured sample dilation during a cooling sequence that formed first the heptahydrate and then the decahydrate [40] , [45] . These results showed that the most important strains were suffered when mirabilite was formed. Such results agree with independent experiments following different experimental protocols [49] , [50] . In the later case, it was also shown that the sample deformation could be quantitatively related to the thenardite equilibrium hypothesis. This states that, provided that thenardite is available in the system when mirabilite is formed, then the solution concentration can be determined by the solubility of thenardite [38] , [39] . With this it is possible to determine the supersaturation with respect to mirabilite and calculate the crystallization pressure. In our analysis of the sodium sulfate test, we used this hypothesis. In support of this choice, it should also be mentioned that there is presently only one study (using hard synchrotron X-rays) directly examining which phase forms during the impregnation cycle [40] . Thermodynamic control over crystallization pressure By carrying out this experiment at different impregnation temperatures (3, 10, 20 and 25 °C), the crystallization pressure and, consequently, the severity of the damage can be varied [32] . 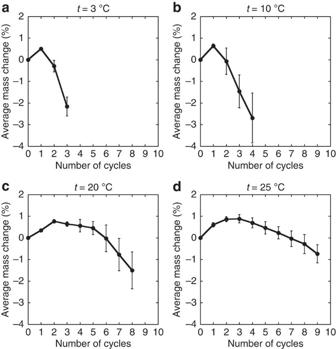Figure 3: Mass change of Portland limestone samples along cycles of sodium sulfate tests. The tests were performed at 3 (a), 10 (b), 20 (c) and 25 °C (d) with a 6.1% (w/w) aqueous solution. The error bars correspond to one s.d. Six samples were used for the tests at 10, 20 and 25 °C, and eight were used for those at 3 °C. Figure 3 shows that samples initially gain mass as they accumulate salt and then lose mass as they are damaged. Figure 3: Mass change of Portland limestone samples along cycles of sodium sulfate tests. The tests were performed at 3 ( a ), 10 ( b ), 20 ( c ) and 25 °C ( d ) with a 6.1% (w/w) aqueous solution. The error bars correspond to one s.d. Six samples were used for the tests at 10, 20 and 25 °C, and eight were used for those at 3 °C. Full size image Mass loss begins after fewer cycles at low temperatures because the solubility difference between mirabilite and thenardite is greatly increased, which raises the supersaturation [38] . The corresponding crystallization pressure is [41] : where R is the gas constant, T is the absolute temperature, is the molar volume of mirabilite. K sp,T and K sp,M are the thermodynamic solubility products of thenardite and mirabilite, respectively. RH sat,T is the deliquescence relative humidity of thenardite and is determined from the water activity in a non-ideal solution calculation using Pitzer coefficients suited for particularly high concentrations [41] . Poro-mechanical stress analysis and damage criterion With Equation (1), it is possible to quantify the variation of crystallization pressure with temperature ( Supplementary Fig. 1 ). However, the corresponding stress is only felt at the pore scale [16] and a macroscopic tensile stress must be calculated to assess possible damage to the porous host [8] , [51] . For this, a poromechanic approach is used [51] , assuming that mirabilite is homogeneously distributed throughout the sample. Averaging the stress over a representative volume element gives the macroscopic tensile stress, σ *: where b is the Biot coefficient, S c is the volume fraction of the pore space filled with crystals and σ r ≅ Δ P C is the radial compressive stress [31] . For Portland limestone, a Biot’s coefficient of 0.74±0.03 is obtained for a porosity of 20±1% and the relation proposed by Fabre and Gustkiewicz [52] for limestones. Increasing the number of cycles, i , increases S c as: where is the molar volume of thenardite, M T is the molar mass of thenardite and is the concentration of sodium sulfate in the solution expressed in g ml −1 . At a concentration of 6.1% (w/w), full saturation is reached between the 11th and the 12th cycles, regardless of the stone porosity ( Supplementary Fig. 2 ). A full derivation of Equation (3) is presented in Supplementary Note 1 . Equations (1, 2, 3) quantify the increase in stresses with decreasing temperature and increasing number of cycles. Maximum values are reached in cycle 12 when the samples completely filled with mirabilite ( Supplementary Fig. 3 ). Using a strain energy criterion, the material is expected to fail if σ * exceeds a critical stress [53] : , where ν ≈0.26 (ref. 54 ) is Poisson’s ratio and σ T is the tensile strength (2.7±0.6 MPa). These values suggest that damage should develop once the stress exceeds . To compare this prediction with experiments, the onset of damage is defined as the cycle at which at least 50% of the samples have begun to lose mass ( Supplementary Fig. 4 ). 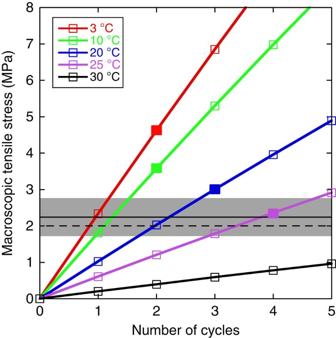Figure 4: Evolution of the predicted macroscopic tensile stress along cycles of impregnation and drying. In each series, the filled symbol indicates the cycle number at which 50% of the samples have lost mass. The dashed line is the maximum stress that could be reached at 30 °C, a temperature at which no damage was observed32. The continuous horizontal line is the critical macroscopic tensile stress as calculated from the average value resulting from the uniaxial tensile strength tests, carried out on 6 samples. The grey-shaded band indicates that value±one s.d. Figure 4 shows that, at temperatures from 3 to 25 °C, this systematically happens (filled symbols) in the first cycle for which the stress exceeds the predicted value. This graph also explains Price’s observation [32] that Portland limestone does not fail at 30 °C, as we find that the maximum value of σ * at that temperature is only 2.0 MPa (discontinuous line). To further check our damage prediction criterion, an additional experiment was performed using a more dilute solution (2% (w/w)) at 10 °C ( Supplementary Fig. 5 ). In this case, instead of having damage initiated between the first and second cycles, it begins between the second and the third cycles, which matches the theoretical prediction. Figure 4: Evolution of the predicted macroscopic tensile stress along cycles of impregnation and drying. In each series, the filled symbol indicates the cycle number at which 50% of the samples have lost mass. The dashed line is the maximum stress that could be reached at 30 °C, a temperature at which no damage was observed [32] . The continuous horizontal line is the critical macroscopic tensile stress as calculated from the average value resulting from the uniaxial tensile strength tests, carried out on 6 samples. The grey-shaded band indicates that value±one s.d. Full size image By allowing systematic variation of the crystallization pressure and the volume fraction of pores filled with salt, the selected experiments establish a damage failure criterion based on strain energy. In our experiments, the initiation of damage is determined on the basis of the initiation of mass loss. Knowledge of the accumulated amount of salts and the crystallization pressure led to reliable prediction of the onset of damage (also highly reproducible, as shown in Supplementary Figs 6–9 ). This failure criterion has been validated using strength data obtained from tests in which the sample fails from the largest flaw that is present. Therefore, it predicts the threshold for failure of flaws of that size. As the stress increases in succeeding cycles, smaller and smaller flaws will grow and cause additional damage. Such small flaws may progressively grow from cycle to cycle owing to fatigue until they are critical and also contribute in failure. This represents the first direct and demonstrated prediction of the onset of damage due to salt crystallization. Of course, conditions in the field are far more complicated than the test we have analysed, with salts entering via rising damp, reactions with atmospheric pollution, deposition of marine salts or microbial activity, and water entering from the soil or precipitation. This means that prediction of damage for a monument requires consideration of the transport processes that bring water and salt to the pores. The complexity of achieving such a prediction is probably one of the reasons why some authors have questioned the usefulness of single-variable controlled experiments in being able to predict outcomes of real-world weathering [55] , [56] . However, while single parameter studies are certainly not sufficient, our study demonstrates how fundamental principles can be used to predict the onset of damage, and emphasizes the importance of transport modelling for achieving similar predictions in real-life exposure. Mass measurements On the lines of the measurements obtained at the British Research Establishment and reported by Price [32] , we carried out measurements of mass changes on 2 × 2 × 2 cm 3 samples of Portland limestone (purchased from Portland Stone Firms Ltd., Portland, Dorset, UK) as a function of cycles of vacuum impregnation with 6.1% (w/w) sodium sulfate solution and drying at 105 °C (18 h long). In a Vötsch VC 4060 climatic chamber (Vötsch Industrietechnik GmbH, Balingen-Frommern, Germany), after 2 h of equilibration at the impregnation temperature (3, 10, 20 or 25 °C) and 0.5 h of evacuation in a glass desiccator, samples were impregnated for 1 h. The stone was cut from several blocks and the resulting samples were randomized to eliminate possible effects of spatial variability, even though this stone is known to be very homogenous [54] . Mass measurements were carried out with a Mettler-Toledo PM4000 technical balance (Mettler-Toledo GmbH, Greifensee, Switzerland) after letting the samples equilibrate in a climatic room at 20 °C and 50% relative humidity for 2 h. When a higher precision was necessary, a Mettler-Toledo NewClassic MS-204S analytical balance was used. Between 3 and 25 °C, a solution with a sodium sulfate concentration of 6.1% (w/w) corresponds to a concentration [57] of 0.0645±0.0001, g ml −1 , whereas the one at 2% (w/w) corresponds to a concentration of 0.02036±0.00003, g ml −1 . Mechanical measurements The direct tensile strength tests were performed on a 10-kN universal testing machine 1454 by Zwick GmbH (Ulm, Germany) on six stone cylinders with a diameter of 2 cm, which were previously vacuum impregnated for 1 h with a 6.1% (w/w) sodium sulfate solution at 20 °C. The used load cell was a 10-kN one. The software for data acquisition was TestXpert II by Zwick. In addition, we performed indirect tensile tests using the Brazilian test on 2 × 2 × 2 cm 3 stone cubes with the same equipment used for the tensile strength tests. The value of 5.8±0.4 MPa (obtained with five samples) is about two times larger than direct tensile strength tests, which is in agreement with what is reported in literature [58] . Reproducibility At each temperature we used groups of six to eight samples (six at 10, 20 and 25 °C; eight at 3 °C). These were cut from the different blocks and randomized to cancel out the possible effect of spatial distribution. In addition, to assess the reproducibility of this procedure we tested two additional groups of six samples, one at 3 °C and one at 20 °C. Results show a very good reproducibility between sample sets in terms of average mass loss and fraction of damaged samples, as shown in Supplementary Figs 6–9 . How to cite this article: Flatt, R. J. et al. Chemomechanics of salt damage in stone. Nat. Commun. 5:4823 doi: 10.1038/ncomms5823 (2014).